Differentiating moss from higher plants is critical in studying the carbon cycle of the boreal biome The satellite-derived normalized difference vegetation index (NDVI), which is used for estimating gross primary production (GPP), often includes contributions from both mosses and vascular plants in boreal ecosystems. For the same NDVI, moss can generate only about one-third of the GPP that vascular plants can because of its much lower photosynthetic capacity. Here, based on eddy covariance measurements, we show that the difference in photosynthetic capacity between these two plant functional types has never been explicitly included when estimating regional GPP in the boreal region, resulting in a substantial overestimation. The magnitude of this overestimation could have important implications regarding a change from a current carbon sink to a carbon source in the boreal region. Moss abundance, associated with ecosystem disturbances, needs to be mapped and incorporated into GPP estimates in order to adequately assess the role of the boreal region in the global carbon cycle. The boreal biome accounts for 7% of global plant biomass and 50% of the global belowground organic carbon pool [1] , [2] . A recent study suggests that boreal forests in the northern high latitudes have sequestered about 0.5 Pg C per year since 1990, which represents a significant portion of the estimated ~1.0 Pg C per year global net forest sink [3] . Moreover, climatic changes associated with increasing atmospheric CO 2 may be greatest at high latitudes [4] , and these changes may have important ramifications for the boreal biome, which may in turn influence the rate of regional and global climatic changes [5] . Therefore, understanding and quantifying the spatial and temporal changes of carbon fluxes over the boreal biome is a high priority. Vegetation gross primary production (GPP) is the largest terrestrial carbon flux and one of the major components controlling land–atmosphere CO 2 exchange. A small error in simulating vegetation production can substantially alter the magnitude of the estimated global carbon balance [6] . Previous studies showed wide and inconclusive results regarding vegetation production over the high-latitude boreal biome. Globally, a comparison of 15 models showed the largest model differences in the boreal region (that is, boreal woodlands and boreal forests) [7] . Model estimates of GPP for boreal North America varied between 2.6 and 11.6 Pg C per year, a larger range than that of temperate North America [8] . Estimates of net primary production (NPP) in Canada’s boreal forest also showed a large uncertainty, varying from 140 to 444 g C m −2 per year from three studies [9] , [10] , [11] . Independently or as part of integrated ecosystem models, the satellite-based light use efficiency (LUE) approach has been used to estimate GPP and NPP at various spatial and temporal scales (see Methods). A recent study showed that an LUE model (the EC-LUE model) substantially overestimates vegetation primary production at young stands because it neglects the impacts of mosses [12] . Mosses often dominate the ground cover and contribute substantially to the satellite signals from young stands [13] . On the other hand, mosses with low LUE are fundamentally different from vascular plants with respect to vegetation production [14] . However, almost all satellite-based models do not explicitly consider the impact of disturbance regimes on vegetation composition of the northern ecosystems, which may cause errors in the application of models using remotely sensed data for the boreal biome. High-quality GPP estimates (using the semi-empirical flux-partitioning algorithm) from the global network of eddy covariance (EC) flux towers make it possible to test the adequacy of algorithms for estimating GPP over large areas. 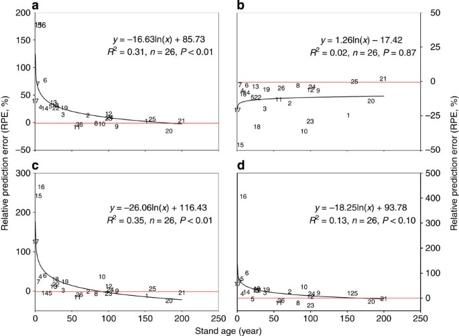Figure 1: The RPE of LUE models versus stand age. (a) The correlation relationship between stand age and RPE of EC-LUE, (b) EC-LUE-2p, (c) MODIS-GPP and (d) CASA models at all sites. Numbers within the graphs are site IDs (Supplementary Table 1). In this study, we test the performance of three LUE models for predicting GPP (EC-LUE, MODIS-GPP and CASA) [12] , [15] , [16] at 26 EC flux towers in the boreal regions of North America, Europe and Asia ( Supplementary Table 1 ; Supplementary Note 1 ), and quantify the relative contribution of different vegetation compositions to ecosystem GPP. The results show that three LUE models overestimate GPP at most sites, especially in younger stands. By separating the LUE and the relative contributions of mosses and vascular plants to the satellite signal using age information, the revised EC-LUE model successfully predicts GPP at all sites. Our regional results show that GPP has been substantially overestimated for the Canada boreal biome by the three LUE models that do not consider the impacts of moss. These results highlight the need to account for the impacts of moss on GPP across the boreal biome in models of terrestrial carbon dynamics. Overestimated GPP over the boreal biome EC-LUE, MODIS-GPP and CASA explained about 68, 42 and 43% of the variation, respectively, of site-averaged GPP over their study periods across all sites ( Supplementary Fig. 1a,c,d ; see Methods). The relative predictive errors (RPEs, see Methods) from the three models decreased with stand age, and prediction errors approached zero for forests older than 50 years ( Fig. 1a,c,d ). All three models overestimated GPP at young forest sites. For example, in forests younger than 50 years, averaged RPE of the EC-LUE, MODIS-GPP and CASA models were 58, 61 and 67%, respectively ( Fig. 1a,c,d ). However, the three models offered accurate predictions for the old forest sites where the RPE was lower than 30% ( Fig. 1a,c,d ). Figure 1: The RPE of LUE models versus stand age. ( a ) The correlation relationship between stand age and RPE of EC-LUE, ( b ) EC-LUE-2p, ( c ) MODIS-GPP and ( d ) CASA models at all sites. Numbers within the graphs are site IDs ( Supplementary Table 1 ). Full size image Differentiation of moss from vascular plants We hypothesize that the overestimation of GPP, especially at young stands, was caused by the presence of moss and the lack of distinction between moss and higher plants in the satellite-derived normalized difference vegetation index (NDVI) data. Moss, one of the major groups of bryophytes, is a ubiquitous and dominant component of ground-level vegetation in the boreal biome. Moss is typically among the first ground layer species to become established after disturbance [17] . For example, at a study site in Interior Alaska, 70% of the surface was covered by moss, and only 30% of the surface was covered by grasses and deciduous shrubs 3 years after fire [18] . Boreal forests are relatively open due to narrow tree crowns and low stand density of dominant trees; as a result, moss can substantially contribute to measured satellite signals [19] . This contribution from moss can be illustrated using a chronosequence of seven adjacent sites recovering from fire disturbances [20] . 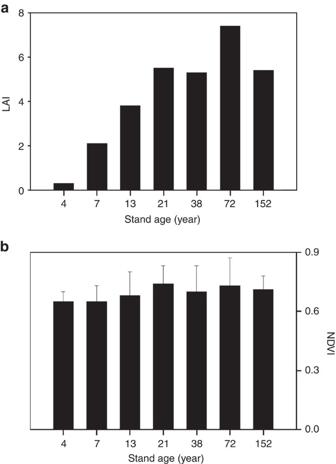Figure 2: Comparison of satellite NDVI field-measured LAI of vascular plants. (a) Comparison of field-measured LAI of vascular plants at seven adjacent sites in Canada; (b) comparison of MODIS NDVI at these seven sites. The sites (and ages in 2002) were CA-NS7 (4 years), CA-NS95 (7 years), CA-NS6 (13 years), CA-NS5 (21 years), CA-NS3 (38 years), CA-NS2 (72 years) and CA-NS1 (152 years). LAI of vascular plants was measured before the end of the growing season in 2004. NDVI values represent the mean NDVI values from May to September during 2002–2006, and the error bars indicate s.d. (see Methods). Figure 2 shows the leaf area index (LAI) of the vascular plants measured from the ground at these sites and their NDVI values derived from satellite data. NDVI includes the greenness contribution from both vascular plants and moss (see Methods). Measured LAI of vascular plants from the ground varied from 0.3 to 7.4 m 2 m −2 across these sites ( Fig. 2a ). In contrast, the NDVI values varied around 0.7, showing small differences across these seven sites ( Fig. 2b ), suggesting all these forests had a closed canopy [21] . The low LAI values in the young stands clearly indicated that their canopies were open. The discrepancy between field-based LAI measurements of vascular plants and satellite-derived NDVI suggests substantial contribution of moss to the satellite signal NDVI in the young stands. Figure 2: Comparison of satellite NDVI field-measured LAI of vascular plants. ( a ) Comparison of field-measured LAI of vascular plants at seven adjacent sites in Canada; ( b ) comparison of MODIS NDVI at these seven sites. The sites (and ages in 2002) were CA-NS7 (4 years), CA-NS95 (7 years), CA-NS6 (13 years), CA-NS5 (21 years), CA-NS3 (38 years), CA-NS2 (72 years) and CA-NS1 (152 years). LAI of vascular plants was measured before the end of the growing season in 2004. NDVI values represent the mean NDVI values from May to September during 2002–2006, and the error bars indicate s.d. (see Methods). Full size image Field experiments indicate that the LUE of moss is only about 10 to 50% of that of vascular plants [22] . To our knowledge, the lower photosynthetic capacity of moss has never been explicitly considered in any of the previous efforts in estimating GPP in the boreal biome. The importance of treating moss and vascular plants separately in estimating GPP can be demonstrated at site and regional scales using a modified EC-LUE model. We revised the EC-LUE model to explicitly include two contributions to ecosystem GPP: one from moss and the other from vascular plants (referred to as the EC-LUE-2p model hereafter). Intrinsic potential LUE values were specified for moss and vascular plants. In addition, we used K_NDVI (see Methods) to represent the fractional contribution of moss to the NDVI signal at the ecosystem level. K_NDVI, the only undetermined parameter of the EC-LUE-2p model, was inverted at the 26 flux tower sites against GPP estimates. Results show that after splitting the EC-LUE model into two parts, the GPP estimates were improved at the 26 flux tower locations and the mean absolute RPE decreased from 32 to 11% across these sites ( Supplementary Figs 1, 2, 3 and 4 ). We found that the contribution of moss to the satellite greenness signal (K_NDVI) was large in newly disturbed young forests, but the signal decreased exponentially with forest age ( Fig. 3 ). 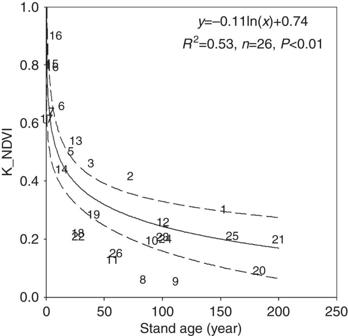Figure 3: The contribution of moss to NDVI versus stand age. K_NDVI indicates the contribution of moss to the NDVI signal. Numbers in the graph are site IDs (Supplementary Table 1). The solid line and equation indicate the regression relationship between stand age and K_NDVI. The two dashed lines indicate the 95% confidence band, and the regression equations arey=−0.11ln(x)+0.84 (high) andy=−0.106ln(x)+0.64 (low). Figure 3: The contribution of moss to NDVI versus stand age. K_NDVI indicates the contribution of moss to the NDVI signal. Numbers in the graph are site IDs ( Supplementary Table 1 ). The solid line and equation indicate the regression relationship between stand age and K_NDVI. The two dashed lines indicate the 95% confidence band, and the regression equations are y =−0.11ln( x )+0.84 (high) and y =−0.106ln( x )+0.64 (low). Full size image Independent field measurements of moss abundance also support the conclusion that the contribution of moss to the satellite greenness signal (K_NDVI) decreases as forests age. A previous study along a wildfire chronosequence found that the bryophyte total cover was inversely correlated with forest age with higher cover in young stands [23] . In Alaskan forests, moss cover showed a unimodal distribution with time since fire occurrence, peaking 30–70 years post fire at the permafrost sites and 5–15 years at the permafrost-free sites [24] . The moss contribution to the NDVI signal is similar to the reported trend, which provides independent validation of the K_NDVI derived from this study. Moreover, the partitioning of GPP between moss and vascular plants by the EC-LUE-2p model matched well with the observations at seven fire chronosequence sites [20] ( Supplementary Fig. 5 ). Impacts on regional GPP estimations Using the improved EC-LUE-2p model (see Methods), the relationship between the contribution of moss to the NDVI signal and forest age derived from 26 flux tower locations ( Fig. 3 ), and the spatial distribution map of forest age [25] , we estimated GPP to be 2.44 Pg C per year for the Canadian boreal biome ( Fig. 4c ; see Methods). Moreover, we quantified the uncertainty of regional GPP estimations resulting from the relationship between stand age and K_NDVI, shown in Fig. 3 (see Methods). The EC-LUE-2p GPP estimates varied from 2.15 to 2.67 Pg C per year over the entire study area for a 95% confidence limit ( Fig. 4a,b ). 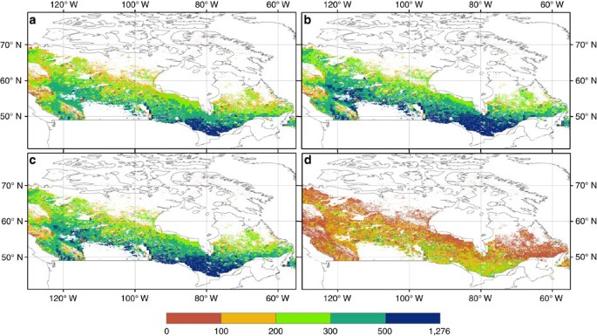Figure 4: Regional GPP estimates of LUE models. (a) The lowest, (b) the highest and (c) mean values of GPP estimates considering the impacts of moss based on the EC-LUE-2p model. (d) The difference in GPP simulations between the original EC-LUE and the EC-LUE-2p models (mean values). The low and high estimates represent the EC-LUE-2p estimates with 95% confidence. The original EC-LUE model does not consider the impacts of moss. The unit of GPP is g C m−2per year. Figure 4: Regional GPP estimates of LUE models. ( a ) The lowest, ( b ) the highest and ( c ) mean values of GPP estimates considering the impacts of moss based on the EC-LUE-2p model. ( d ) The difference in GPP simulations between the original EC-LUE and the EC-LUE-2p models (mean values). The low and high estimates represent the EC-LUE-2p estimates with 95% confidence. The original EC-LUE model does not consider the impacts of moss. The unit of GPP is g C m −2 per year. Full size image In comparison, EC-LUE, MODIS-GPP and CASA generated estimates of 3.30, 3.69 and 3.98 Pg C per year, respectively, for the same region when moss contribution was not explicitly considered. This finding represents an overestimation of 34–63% of the result from the EC-LUE-2p model ( Fig. 4d ). The EC-LUE-2p-simulated average GPP was 388 g C m −2 per year; even the maximum estimation of GPP was 425 g C m −2 per year, substantially lower than the 601 g C m −2 per year recently obtained over the global boreal biome by diagnostic models [26] . This result clearly demonstrates the importance of moss, disturbance and forest development stage in estimating vegetation production in the boreal biome. GPP is a critical component of the carbon cycle because it signifies carbon uptake by ecosystems. GPP estimates have been directly or indirectly used to evaluate regional carbon budgets [27] . For example, GPP maps were used to provide prior information for atmospheric inversion experiments [28] , and studies have shown inverse estimates of CO 2 fluxes in boreal Asia to be very sensitive to these prior estimates [29] . Unfortunately, spatial patterns of the contributions from moss and/or vascular plants to satellite signals have never been separately mapped and used in any of the previous efforts to estimate regional GPP. Consequently, current estimates of regional GPP are likely much higher than reality, as the photosynthetic capacity of moss is implicitly and artificially elevated to the same level as that of vascular plants. The northern latitude boreal biome is generally considered to be acting as a considerable sink for atmospheric CO 2 based on the results from both ‘top-down’ and ‘bottom-up’ approaches [30] . However, the precise role that the northern high-latitude region plays in the global carbon budget is not well understood because of model uncertainties [31] . For example, a study based on a nested inverse modelling system indicates Canada’s sink to be large (0.34±0.14 Pg C per year) [28] . However, ecosystem modelling and inventory-based analysis found Canada’s forest to be a weak sink of 0.05–0.07 Pg C per year [11] , [25] . Regional carbon balance strongly depends on the accuracy of estimated GPP. An overestimation of regional GPP, as we have found in this study, has important ramifications for the carbon cycle in the boreal region. Although we only examined LUE models in this study, the conclusion is applicable to GPP models based on enzyme kinetics. A recent study reported large differences in enzyme kinetics between moss and vascular plants [32] . Moreover, the satellite-based LAI was used to drive physiological models. For example, GPP simulations from the Breathing Earth System Simulator, which integrates the MODIS LAI product with the enzyme kinetics model to estimate GPP, were most sensitive to LAI [33] . However, these physiological models did not differentiate the different contributions of moss and higher plants to satellite signal and ecosystem GPP. Therefore, this study highlights the importance of incorporating distinct structural and functional properties of ecosystems into regional modelling frameworks. The implication of the results from this study to the total carbon budget of the boreal biome is important but quantitatively unknown as carbon sinks and sources are determined by both GPP and respiration. Given that plant autotrophic respiration (Ra) is proportional to GPP (about half) [34] for both moss and vascular plants [35] , previous Ra estimates are likely proportionally overestimated. However, Ra overestimates could not offset all GPP overestimates as the proportionality is about half, and the remaining half would result in overestimates of NPP (GPP minus Ra). The impacts of failing to account for the presence of moss on heterotrophic respiration are difficult to evaluate because heterotrophic respiration is affected by many processes, including NPP allocation among moss and higher plants and mortality; we do not yet have a model that comprehensively represents all these processes mechanistically. Nevertheless, some rough estimation can illustrate the consequence of GPP overestimates on the regional carbon budget. Assuming that the overestimated NPP is half of the overestimated GPP and is either completely returned to the atmosphere via heterotrophic respiration (low impact of GPP overestimation) or entirely accumulated in terrestrial ecosystems (high impact of GPP overestimation), the net impact on net carbon gain would range from 0 to 0.43 (EC-LUE), 0 to 0.62 (MODIS-GPP) and 0 to 0.77 Pg C per year (CASA) according to the GPP differences between EC-LUE-2p and these models. It is not likely that all overestimated NPP using the conventional approaches would be respired via heterotrophic respiration or completely retained by the ecosystems; the correct answer probably falls in the middle. If these considerations were incorporated in previous carbon sink estimates [25] , [28] , Canadian forests could be a source rather than a sink. In summary, the impacts of failing to differentiate the contributions of mosses and higher plants to the carbon cycle are substantial. Future research on the impact of moss on the carbon cycle, especially ecosystem respiration, is needed to reduce the uncertainty in estimating the regional carbon sink strength. Our results suggest that characterizing plant composition and percent cover of bryophytes in the boreal biome is critical for quantifying the impacts of land surface dynamics on climate change because the boreal biome is the second largest biome in the world [36] . Bryophytes play an important role in ecosystem structure and function of boreal forests and have a profound impact on terrestrial carbon, water and nutrient budgets [37] . The importance of bryophytes and the lack of capability in mapping their dynamics thus highlight the need to develop remote sensing approaches to quantify the composition and percent cover of bryophytes in the region [13] . Even though MODIS data are gridded, the sensor flies over a given point on the ground at different angles over time. Therefore, in theory, the contribution of K_NDVI should be different depending on the off-nadir view angle. This would change the MODIS observation for each orbit but it might also be a chance to estimate the fractional contribution of mosses across the landscape. Several studies found that satellite observations from multiple view angles significantly improve the assessment of vertical vegetation structure [38] , [39] . At the same time, off-nadir view angles minimize distorting background/understory effects and provide new information for separating the spectral contribution of the forest floor (or understory layer) from the tree canopy layer [40] . Moreover, field manipulative experiments are needed to actually measure the contribution of bryophytes to satellite signals at the local scale, which will improve our understanding of the function of bryophytes. Our current understanding of moss photosynthetic capability is still very limited. For example, the value of 0.64 g C m −2 MJ −1 absorbed photosynthetically active radiation (APAR) for potential LUE of moss used in this study was 30% that of vascular plants according to currently available studies [14] . A previous study showed that the net CO 2 uptake rates of mosses were only about 10–40% those of vascular plants on a dry mass basis [41] . Similarly, the LUE of moss in Alaskan tundra was about 18% that of the overstory canopy [42] . Apparently, more comparative studies on photosynthetic capacity and LUE of mosses and vascular plants are needed to further improve our understanding of the role of mosses in regional and global carbon cycles. In addition, we lumped and did not differentiate the vascular plants (for example, shrubs and grasses) covering the ground of boreal forests from the trees in this study, as no systematic differences in photosynthetic capacity or LUE have been reported between these life forms. Nevertheless, understanding the importance of the contribution of ground vascular plants to the satellite signals in these forests versus their productivity and their contribution to ecosystem GPP can shed useful light to ecosystem carbon dynamics as the composition of these life forms changes over time [18] . In this study, we found substantial impacts of disturbances on ecosystem structure and composition and their subsequent impacts on ecosystem productivity in boreal ecosystems. Disturbances alter forest structure and vegetation composition and cause higher bryophyte cover in young stands [23] . Increasing temperature in the northern high latitudes has resulted in well-documented increases in frequency, intensity, seasonality and extent of various disturbances such as fire and insect outbreaks, and these trends are likely to continue with warming and drying [43] . The impacts of stand-replacing disturbances such as fire and harvesting might have been underestimated in the past, which can alter the forest age structure and contribution of moss to ecosystem GPP. It is imperative to incorporate these structural and functional changes of ecosystems into regional modelling frameworks to adequately assess the impacts of disturbances on the carbon cycle and global climate. LUE model Predicting the GPP of terrestrial ecosystems has been a major challenge in quantifying the global carbon cycle [44] . Among predictive methods, the LUE model may have the greatest potential to adequately address the spatial and temporal dynamics of GPP because of its theoretical basis and practicality [45] . The LUE model is built on two fundamental assumptions [46] : (1) the ecosystem GPP is directly related to APAR through LUE, where LUE is defined as the amount of carbon produced per unit of APAR, and (2) realized LUE may be reduced below its theoretical potential value by environmental stresses, such as low temperatures or water shortages [47] . The general form of the LUE model is where fPAR is the fraction of PAR absorbed by the vegetation canopy, PAR is the incident photosynthetically active radiation (MJ m −2 ) per time period (for example, day or month), ε max is the potential LUE (g C m −2 MJ −1 APAR) without environmental stress, f is a scalar varying from 0 to 1 that represents the reduction of potential LUE under limiting environmental conditions, and the multiplication of ε max and f is realized LUE. Numerous studies have developed various LUE models such as the CASA model [16] . In this study, three LUE models including MODIS-GPP, CASA and EC-LUE, which have been widely validated and applied at global scales, were selected to examine the impact of moss on estimating vegetation GPP in the boreal forest biome. MODIS-GPP product The MODIS-GPP algorithm is an LUE-based model, with inputs from MODIS LAI/fPAR (MOD15A2), land cover and biome-specific climatological data sources from the National Aeronautics and Space Administration (NASA) Data Assimilation Office [15] . LUE is calculated based on two factors: the biome-specific potential LUE ε max , a multiplier that reduces the LUE when cold temperatures limit plant function, and a second multiplier that reduces the potential LUE when vapour pressure deficit (VPD) is high enough to inhibit photosynthesis. It is assumed that soil water deficit covaries with VPD and that VPD will account for drought stress. The GPP algorithm was tested with flux data sets from a range of biomes [48] . CASA model CASA is a LUE model that uses satellite measurements to estimate vegetation NPP [16] . The model directly translates APAR into NPP based on LUE, which is a product of optimal efficiency and the regulatory functions of environmental factors (for example, temperature and water stress). The CASA model directly simulates NPP, and an approximate conversion of 0.47 between NPP and GPP is used in this study [34] . EC-LUE model The EC-LUE model is driven by only four variables: NDVI, PAR, air temperature ( T , °C) and the evaporative fraction [49] . GPP was computed from fPAR, PAR and downregulators. The downregulators represent plant stresses due to suboptimal temperature ( T s ) and water ( W s ). where Min denotes the minimum values of T s and W s , and the impacts of temperature and moisture on LUE were assumed to follow Liebig’s Law (that is, LUE is only affected by the most limiting factor at any given time). T min , T max and T opt are the minimum, maximum and optimum air temperatures (°C) for photosynthetic activity, respectively. If air temperature falls below T min or increases beyond T max , T s is set to zero. In this study, T min and T max were set to 0 and 40 °C, respectively, whereas T opt was set to the mean temperature during the growing season. LE is the latent heat (MJ m −2 ), and MODIS-ET was the product used in this study. R n is the net radiation (MJ m −2 ). EC-LUE-2p model To investigate the impact of moss on estimations of ecosystem GPP, we developed the EC-LUE-2p model by separating vegetation production into two components based on the EC-LUE model: vascular (GPP v ) and moss (GPP m ): where ε vmax and ε mmax are the potential LUE of vascular and moss plants, respectively. In this study, ε vmax is set at 2.14 g C m −2 MJ −1 APAR [12] , [50] , and ε mmax is assumed to be 30% of ε vmax or 0.64 g C m −2 MJ −1 APAR based on previous studies [14] , [41] , [42] . K_NDVI indicates the proportional contribution of moss to the NDVI signal; PAR v and PAR m are the total photosynthetically active radiation partitioned to the vascular and moss plants, respectively. The calculations of fPAR, W s and T s are reported in equations (3), (4) and (5). We used the Beer–Lambert law to exponentially partition PAR between the vascular and moss surface: where k is the light extinction coefficient ( k =0.5). LAI is MODIS LAI data, and the proportional contribution of vascular plants to the LAI signal is assumed to be the same as that of NDVI. The linear relationship between NDVI and fPAR was used in EC-LUE, which was supported by many studies [50] , [51] . The strong linear relationship of NDVI and fPAR, derived from a total of 16 plant species of annuals, vines, deciduous and evergreen shrubs and trees, was used in our model [52] . Strong linear relationships between NDVI and field-measured fPAR were also observed at high-latitude ecosystems [53] , [54] . Moreover, we compared the MODIS-fPAR product and fPAR calculations based on NDVI in this study, and results showed that they were comparable across almost all sites ( Supplementary Fig. 6 ). The EC-LUE-2p model and our study are built on two facts: first, ecosystem GPP includes contributions from higher plants and moss (K_NDVI was used to represent contributions to the satellite signal from moss in the model). In case of no contribution from moss, K_NDVI would be zero. Second, the intrinsic LUEs of higher plants and moss are different. This difference is the fundamental basis for our ability to separate the contributions of moss and vascular plants. If ecosystem GPP did not perform as highly as expected for vascular plants, it must contain mosses that have a substantially lower photosynthetic capacity. This is the biological foundation of the EC-LUE-2p model. The only unknown in the model is K_NDVI, which can be solved analytically according to equations (6)–(8), , : In reality, K_NDVI is solved statistically using estimates of GPP from EC measurements, as we have done in this study. The biological and physiological bases of the model (two facts described above) and the statistical optimization of K_NDVI against EC measurements strictly and uniquely constrained the meaning of K_NDVI. For the EC-LUE-2p, PAR, R n , T and LAI are model forcing data that can be measured by EC towers and derived from satellite data. Potential LUEs of vascular and moss plants (that is, ε vmax and ε mmax ) are model parameters, which have been determined as mentioned above. The only undetermined parameter is K_NDVI, which is optimized at each EC site against GPP estimates. The regression procedure (Proc NLIN) in the Statistical Analysis System (SAS, SAS Institute, Cary, NC, USA; any use of trade, firm or product names is for descriptive purposes only and does not imply endorsement by the US Government) was applied to optimize the values for K_NDVI at each site. At the regional scale, the relationship between K_NDVI and stand age ( Fig. 3 ) was used to calculate the spatial pattern of K_NDVI, based on the spatial distribution map of forest age in Canada [25] , [55] . We validated this large-scale model application at the site level. First, we used the relationship shown in Fig. 3 for each site individually and calculated K_NDVI to simulate GPP. Second, the correlation relationship between K_NDVI and stand age was recalculated by excluding a given site, and the relationship was used to estimate K_NDVI and GPP at this site. Simulations of GPP at these two schemes were then compared with observations. The results showed good model performance using the relationship between K_NDVI and stand age ( Supplementary Fig. 7 ). Model operation and forcing data at the EC sites The EC-LUE and CASA models were run at 8-day time steps at the EC sites. Environmental variables measured at the EC sites were used to drive these two models. The 8-day NDVI data with 1-km spatial resolution (MOD13) were retrieved at the EC sites. MOD13 has a quality control (QC) layer to indicate data reliability for each pixel (good data, marginal data, snow/ice, cloudy and missing). In this study, we considered NDVI data with a ‘marginal’ or ‘cloudy’ QC flag to be unreliable. We temporally filled the missing or unreliable NDVI at each 1-km MODIS pixel based on its corresponding quality assessment data field [56] . First, if the first (or last) 8-day NDVI value is unreliable or missing, it will be replaced by the closest reliable 8-day value. Second, other unreliable NDVI will be replaced by linear interpolation of the nearest reliable value before it and the closest reliable value after it. If there are no reliable NDVI values during the entire year, the annual maximum NDVI will be chosen from unreliable periods in the current year and will be used as a constant value across the entire year. The 8-day MODIS evapotranspiration (ET) data (MOD16) [57] at 1-km spatial resolution was used to indicate actual ET, and potential ET (PET) was calculated by the method of Thornthwaite [58] . The 8-day MODIS-GPP product (MOD17) data at 1-km spatial resolution were used to examine MODIS-GPP algorithm verification at the EC sites. The same method that was used for NDVI was used to conduct data QC and fill missing data gaps for MODIS-ET and -GPP products. Statistical analysis Three metrics were used to evaluate the performance of the four models in this study: the coefficient of determination ( R 2 ), absolute predictive error (PE) and RPE. PE quantified the difference between simulated and observed values, and RPE was computed as where and are mean simulated and mean observed values, respectively. Field-measured LAI at seven Canada sites Field-measured LAI of vascular plants at seven adjacent Canada sites recovering from fire disturbances (that is, CA-NS1, CA-NS2, CA-NS3, CA-NS5, CA-NS6, CA-NS95 and CA-NS7) was used to compare with satellite NDVI values. LAI was measured by harvest [20] . The harvests occurred shortly before the end of the growing season in 2004. Moreover, we used 8-day MODIS-NDVI product (MOD13). Figure 2 shows the mean NDVI values from May to September during 2002–2006, and the error bars indicate s.d. Model forcing data over the regional scale We used input data sets of R n , T and PAR from the Modern Era Retrospective-Analysis for Research and Applications (MERRA) [59] archive in 2004 to drive the CASA and EC-LUE models for regional GPP estimation. The MODIS-GPP (MOD17) product was directly used in this study. MERRA is a NASA reanalysis for the satellite era using a major new version of the Goddard Earth Observing System Data Assimilation System Version 5 (GEOS-5), which was used to interpolate and grid these point data at short time intervals, producing an estimate of climatic conditions for the world at 10 m above the land surface (approximating canopy height conditions) and at a resolution of 0.5° latitude by 0.6° longitude. The MERRA reanalysis data set has been validated carefully at the global scale using surface meteorological data sets to evaluate the uncertainty of various meteorological factors (for example, temperature, radiation, humidity and energy balance) [60] . This validation showed that MERRA considerably reduced imbalances in energy and water [61] . Detailed information on the MERRA data set is available at http://gmao.gsfc.nasa.gov/research/merra/ . Eight-day MODIS LAI/fPAR (MOD15), NDVI (MOD13) and ET (MOD16) at 1-km spatial resolution also were used to drive the CASA, EC-LUE and EC-LUE-2p models for estimating regional GPP. The same method as that used at the EC sites was used to conduct data QC and fill missing data gaps for MODIS products. All satellite-based products were resampled at a resolution of 0.5° latitude by 0.6° longitude to match that of the MERRA reanalysis data set. Uncertainty of GPP Estimations Figure 3 shows the correlation between K_NDVI and stand age. To quantify the uncertainty, we calculated the 95% confidence limits of the regression relationship between stand age and K_NDVI. The high and low 95% confidence limits were used to quantify the maximum and minimum GPP estimations, respectively. This study used MODIS NDVI and LAI products of 1-km resolution to estimate regional GPP using the EC-LUE, EC-LUE-2p and CASA models. These products were generated from MODIS surface reflectance after correcting for the effects of cloud contamination, ozone absorption and aerosols, and adjusted to nadir and standard sun angles using bidirectional reflectance distribution function models [62] . A simple linear interpolation method was used to fill unreliable or missing NDVI or LAI data [56] , which may introduce additional uncertainty into our GPP estimation. Moreover, we used the relationship between stand age and contribution of moss to the satellite signal to improve regional GPP estimations. However, we did not consider impacts of other factors on moss fraction cover, such as vegetation, soils and surface water. On the basis of long-term measurement and literature data, synthesis analysis showed substantial differences of moss cover in the uplands and floodplains [63] . How to cite this article: Yuan, W. et al. Differentiating moss from higher plants is critical in studying the carbon cycle of the boreal biome. Nat. Commun. 5:4270 doi: 10.1038/ncomms5270 (2014).